Synthesis ofcis-thiiranes as diastereoselective access to epoxide congeners via 4π-electrocyclization of thiocarbonyl ylides Organochalcogen heterocycles are ubiquitously present and widely utilized in various fields. Among them, oxirane has been extensively studied, and all of the stereoisomeric forms are readily available. In contrast, synthetic studies on thiirane were rarely reported, and thus the useful sulfur-congener of oxirane has been difficult to access in a stereodefined form. In this research, a general stereoselective synthesis of cis -thiiranes is accomplished by taking advantage of stereospecific electrocyclization of trans -thiocarbonyl ylides, which are generated in situ from readily available E , E -aldazine N -oxides upon treatment with Lawesson’s reagent. This newly developed practical method provides a variety of cis −1,2-diarylthiiranes as essentially single diastereomers in high yields under mild reaction conditions. The intermediacy of trans -thiocarbonyl yilde is confirmed by mechanistic experiments, and the excellent stereocontrol is rationalized by DFT calculation. The chalcogens, elements in group 16 of the periodic table, are widely utilized in various fields (Fig. 1a ). In particular, non-covalent interaction between chalcogen atoms and electron donors, so-called chalcogen bonding plays important roles in materials chemistry [1] , [2] , [3] as well as noncovalent organocatalysis [1] , [4] , [5] . Moreover, the combination with other electropositive elements composes chalcogenides, which have numerous applications such as chalcogenide glasses [6] , [7] , [8] , polymer solar cells [9] , wide band gap semiconductors [10] , and electrochemical sensors [11] . Furthermore, chalcogens are often found in natural products and pharmacologically active compounds. Among them, three-membered heterocycles containing a chalcogen are ubiquitous subunits, and significant efforts have been dedicated to the development of synthetic methods for oxiranes [12] , [13] . The sulfur congeners, thiiranes are also useful synthetic precursors that can be transformed into an array of functional groups via ring-opening or desulfurization [14] , [15] , [16] , [17] , [18] , [19] , [20] . In addition, versatile sulfur-containing polymers can be produced via ring-expansion polymerizations or copolymerizations [21] , [22] , [23] , [24] , [25] . Moreover, thiiranes have been examined as analogs of biologically active oxiranes [26] , [27] , [28] , and several derivatives showed inhibitory activity against gelatinases [29] , [30] . However, despite the apparent utility, synthetic methods for thiiranes are not well established compared to oxiranes (Fig. 1b ). Indeed, the stereoselective construction of thiiranes remains a great challenge. For example, whereas all of the stereoisomers of stilbene oxide can be easily prepared and are even commercially available, the related stilbene sulfides are typically produced through stereospecific conversion of the corresponding stilbene oxides [31] . Clearly, it is highly desirable to develop a general and practical stereoselective synthesis of thiiranes. Fig. 1: Thiiranes as synthetic targets. a Importance of organochalcogens. b Comparison between oxiranes and thiiranes. Full size image Thiirane synthesis has been generally accomplished via the conversion from oxirane analogs with thiourea or thiocyanate as a sulfurating reagent (Fig. 2a ) [32] , [33] , [34] , [35] , [36] , [37] , [38] . Consequently, the stereostructure of thiiranes necessarily relies on the configuration of oxiranes. In a special case, it is possible to introduce a stereochemical element during the chalcogen substitution step via a kinetic resolution process as recently demonstrated by the List group utilizing the chiral phosphoric acid catalysis [39] , [40] . However, only terminal thiiranes can be prepared by this strategy. Alternatively, the episulfidation of alkenes has been investigated [15] , but this seemingly straightforward epoxidation-like approach is applicable only to a limited range of cyclic alkenes. Otherwise, stereoselective synthesis of thiiranes has rarely been developed [41] , [42] , [43] , [44] , [45] , and most of the reported examples have serious drawbacks such as low stereoselectivity, narrow substrate scope, and/or the requirement of highly toxic reagents. Among these precedents, a unique synthetic sequence of the Barton–Kellogg reaction is noteworthy (Fig. 2b ) [46] , [47] , [48] , [49] , [50] , [51] , [52] , [53] . The Kellogg group developed a sequential process involving non-stereoselective sulfurization of azines followed by dehydrogenation to furnish thiadiazolines ( 1 ) as a mixture of diastereomers [48] . Interestingly, the isolated trans- and cis- 1 were stereospecifically transformed to the corresponding cis- and trans- thiiranes, respectively. The stereochemical outcome was rationalized by 4π-electrocyclization of the putative thiocarbonyl ylides ( 2 ), which were derived from 1 via thermal extrusion of dinitrogen gas. Unfortunately, despite the intriguing stereochemical properties, this method has not received much attention because of the use of a highly toxic and inconvenient gaseous sulfurating reagent, H 2 S. Moreover, the formation of 1 requires harsh and toxic oxidants such as Pb(OAc) 2 or diethyl azodicarboxylate (DEAD). The most critical drawback is the lack of stereoselectivity in the sulfurization step, which diminishes the practicality of this method quite substantially. Our group has been interested in the unusual reactivity of electrophilically activated 1,2-diazines and related organonitrogen compounds [54] , [55] . While investigating the reactions of aldazine N -oxides ( 5 ) with various electrophiles, we serendipitously observed the highly diastereoselective formation of cis -disubstituted thiiranes ( 6 ) upon treatment with Lawesson’s reagent (LR) (Fig. 2c ). Fig. 2: Approach to stereoselective synthesis of thiiranes. a Common method for thiirane synthesis. b Previous approach to thiiranes via the intermediacy of thiocarbonyl ylides. c This work: Diastereoselective synthesis of cis -thiiranes from aldazine N -oxides. LR Lawesson’s reagent, d.r. diastereomeric ratio. Full size image Herein, we report a general synthetic method for cis- diarylthiiranes through the stereospecific sulfurization of aldazine N- oxides. Our newly discovered process resembles the Barton–Kellogg reaction but exhibits several distinct advantages. Because azine is pre-oxidized under relatively mild conditions [56] , [57] , [58] prior to the sulfurization, harsh oxidation conditions are avoided. In addition, a more convenient and less toxic sulfurating reagent, LR, is utilized. Most importantly, cis -thiiranes are produced with an excellent level of diastereoselectivity. Aldazine N- oxides ( 5 ) were readily prepared by a two-step sequence involving double condensation of aldehydes with hydrazine [59] , [60] and the following N- oxidation (see Section 2.1 of the Supplementary Information for details). [56] , [57] , [58] All of 5 were obtained with E , E -configuration [59] , [60] and are bench-stable solids that can be stored for months without decomposition. On the other hand, it was challenging to access unsymmetrical substrates because of the disproportionation during both C = N condensation and N -oxidation, and aliphatic aldazines are unstable under the N -oxidation conditions. 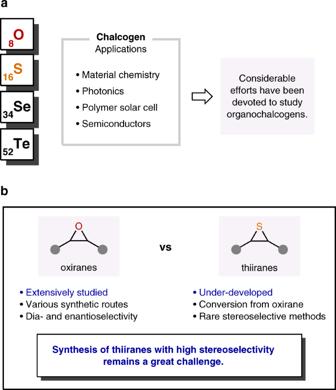Fig. 1: Thiiranes as synthetic targets. aImportance of organochalcogens.bComparison between oxiranes and thiiranes. At the outset, the reaction conditions for thiirane formation were optimized with benzaldazine N- oxide ( 5a ) and LR (Table 1 ). In the presence of 1.0 equiv of LR in CH 2 Cl 2 at −10 °C, 2,3-diphenylthiirane ( 6a ) was produced in 13% yield with a reasonably high 84:16 cis / trans selectivity (entry 1). Although the yield was low, the dominant formation of cis- isomer was encouraging. When the reaction was conducted in polar MeCN, both yield (23%) and cis- selectivity (94:6) were increased (entry 2). Thus, a few other polar solvents were examined. DMSO was unsuitable because it reacted vigorously with LR. Gratifyingly, the use of DMF resulted in a synthetically useful 62% yield with an enhanced 97:3 cis- selectivity (entry 3). The analysis of the crude mixture revealed that a small amount of DMTF was generated by thionation of DMF. Hence, DMTF was employed as a solvent in order to evaluate the potentially promoting activity, but a drastically decreased 25% yield was afforded (entry 4). Subsequently, upon a brief survey of other amide solvents, an improved 67% yield and an excellent 99:1 cis- selectivity were obtained in DMPU (entry 5), whereas the use of DMA was less effective (entry 6). In these experiments, a noticeable exotherm was detected during the addition of LR. It was hypothesized that the elevated internal temperature could have caused unproductive side reactions, leading to moderate chemical yields. Therefore, the reaction was carried out at a lower temperature. For this purpose, DMF was employed as a solvent because of the high melting point of DMPU. At −50 °C, an increased 71% yield was obtained with an essentially exclusive cis- selectivity (entry 7). To our delight, when LR was added slowly as a solution for finer temperature control, the yield was even further improved to 78% (entry 8). In this case, DMPU was used as a solvent for LR because DMF reacts with LR at room temperature [61] . With this protocol, higher and lower loadings of LR were examined, but the yields were slightly diminished in both cases (entries 9 and 10). Table 1 Reaction conditions optimization a Full size table With the optimal reaction conditions in hand, a wide range of 1,2-diarylaldazine N -oxides was surveyed (Fig. 3 ). Electron-withdrawing groups were well tolerated. Not only p -fluorine but also sterically hindering o -chlorine/bromine substituents could be introduced, producing 6b – 6d in 59–73% yields. Moreover, highly electron-deficient, p- trifluoromethyl-substituted thiirane 6e was successfully afforded in 63% yield. It was possible to install electron-donating alkyl groups at any positions on the aryl rings, too. Thiiranes with p- methyl ( 6f ), p - tert -butyl ( 6g ), o -methyl ( 6h ), or m -methyl ( 6i ) groups were formed in 71–91% yields. Strongly electron-donating alkoxy groups could be present at the o -positions, again, without steric encumbrance problem, providing 6j in still high yield and diastereoselectivity. The presence of m -methoxy groups was allowed to give 6k in 71% yield, as well. Unfortunately, p- alkoxy substitution resulted in an unstable product. Even though the predominant formation of 6l was observed by 1 H NMR analysis of the crude mixture, the thiirane decomposed slowly to the corresponding alkene upon purification on silica gel. Thus, 6l was obtained as a mixture with alkene (86:14). Moreover, the loss of sulfur atom took place spontaneously over time to increase the amount of alkene upon storage even in the fridge (Fig. 4 ). [14] This desulfurization process is not stereospecific, and thus a mixture of Z- and E- alkene isomers 7 was produced from an essentially diastereopure thiirane. Such decomposition was suppressed by attenuating the electron-donating ability of the alkoxy group. Hence, 6m containing p -trifluoromethoxy groups could be isolated in 69% yield. Finally, heteroaromatic substrates were examined, and both 3-thienyl and 3-furyl moieties were successfully employed to give 6n and 6o in 64% and 57% yields, respectively. 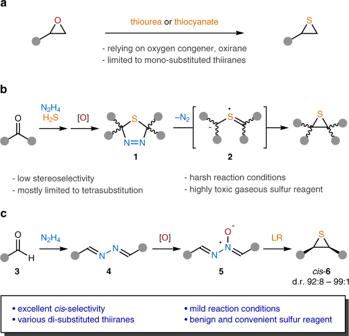Fig. 2: Approach to stereoselective synthesis of thiiranes. aCommon method for thiirane synthesis.bPrevious approach to thiiranes via the intermediacy of thiocarbonyl ylides.cThis work: Diastereoselective synthesis ofcis-thiiranes from aldazineN-oxides. LR Lawesson’s reagent, d.r. diastereomeric ratio. On the other hand, the isomeric 2-thienyl and 2-furyl substrates could not be employed because the corresponding thiirane products decomposed rapidly on silica gel. Overall, cis -diarylthiiranes were consistently obtained in good yields with excellent diastereoselectivity regardless of the electronic and steric properties of the substituents. The cis -configuration of thiirane products was unambiguously established by X-ray crystallographic analysis of 6d (Supplementary Fig. 4 ). Fig. 3: Substrate scope of LR-mediated cis- diarylthiirane synthesis. a Reaction conditions: 5 (1.0 mmol) in DMF (5.0 mL) and LR (1.0 mmol) in DMPU (5.0 mL). Isolated yields after column chromatography are given. Diastereomeric ratio was determined by 1 H NMR analysis of the isolated material. Data after recrystallization are given in the parenthesis. b Contaminated by alkene (86:14). Full size image Fig. 4: Instability of electron-rich thiirane. Non-stereospecific, spontaneous desulfurization of p -alkoxy- cis -thiirane. Full size image Mechanistic experiments were carried out for the newly developed cis- selective thiirane synthesis (Fig. 5 ). 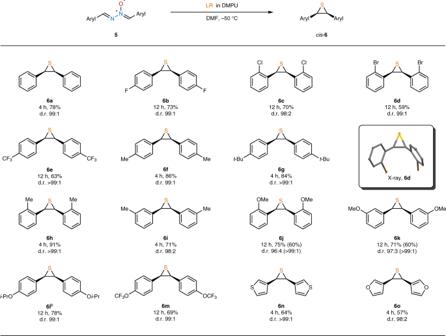Fig. 3: Substrate scope of LR-mediatedcis-diarylthiirane synthesis. aReaction conditions:5(1.0 mmol) in DMF (5.0 mL) and LR (1.0 mmol) in DMPU (5.0 mL). Isolated yields after column chromatography are given. Diastereomeric ratio was determined by1H NMR analysis of the isolated material. Data after recrystallization are given in the parenthesis.bContaminated by alkene (86:14). On the basis of Kellogg’s study [48] , it was hypothesized that the observed cis -configuration of thiiranes would be originated from the intermediacy of a trans- thiocarbonyl ylide via stereospecific conrotatory 4π-electrocyclization. Therefore, trapping of a putative trans- thiocarbonyl ylide 8 was pursued, and the 1,3-dipolar cycloadducts 9a and 9b were successfully obtained employing N- phenylmaleimide and maleic anhydride (Fig. 5a ) [62] . The 1,3- trans -configurations of these compounds were determined by single-crystal X-ray diffraction analysis (Supplementary Figs. 2 and 3 ), highly supporting the presence of trans- 8 . In addition, a crossover experiment was conducted with a 1:1 mixture of 5a and 5f (Fig. 5b ). Under the standard reaction conditions, only 6a and 6f were afforded, and the scrambled product 6af was not detected. Therefore, the intermolecular reaction pathway was excluded. Fig. 5: Mechanistic experiments. a Trapping the trans -thiocarbonyl ylide intermediate with dipolarophiles. b Crossover experiment with two different aldazine N -oxides. Full size image To gain insight into the detailed reaction mechanism, a computational study was performed by the density functional theory calculation at the M06-2X/6-311 + G(d,p)/PCM(DMF) level of theory (Fig. 6 , Supplementary Data 1 ) [63] , [64] , [65] , [66] . Whereas typical thionation with LR requires heating, our thiirane formation proceeds at a subzero temperature. Thus, dissociation of LR is less likely under our reaction conditions, and the dimeric form was employed in the computational analysis. The process is initiated by the coordination of aldazine N -oxide 5a onto dimeric LR to generate Int I [67] , and the subsequent cyclization affords oxathiazaphospholidine sulfide Int II , completing a stepwise formal [3 + 2] cycloaddition [68] . Then, the exergonic production of zwitterion Int III is driven by the formation of a stable P = O bond [67] . Until here, even after cleavage of covalent bonds in the LR moiety, the electron-deficient phosphorus centers and the electron-rich sulfur anions still appear to associate through electrostatic interaction. Notably, a few calculated structures were located only when the solvent effect of DMF was considered in the computation. This result is consistent with the experimental observation. During the reaction conditions optimization, the yield of thiirane was substantially improved upon the use of DMF (Table 1 , entry 3), whereas the reactions in less polar solvents gave inferior results (Table 1 , entries 1, 2, and 4). It is presumed that a highly polar solvent is needed for the stabilization of multiply charge-separated transition structures and intermediates. Subsequently, a facile intramolecular nucleophilic attack of the reactive sulfur anion onto the neighboring diazenium moiety furnishes trans- thiadiazoline Int IV with concomitant release of an oxygenated LR analog 10 . The calculated pathway up to this point from I is composed of a series of stereospecific transformations, all of which take place at one side of 5a . In consequence, the E , E -geometry of aldazine N -oxide leads to the trans -configuration of thiadiazoline. Then, upon a concerted extrusion of dinitrogen gas, the experimentally confirmed trans- thiocarbonyl ylide Int V is produced [69] . Alternatively, Int IV may split into a diazo compound and a thial ( Int V’ ) via a [3 + 2] cycloreversion (red line) [50] . This potential side reaction is endergonic and reversible. Hence, the stereochemical integrity of Int IV may be compromised through unselective recombination. Fortunately, the activation energy of the desired pathway is 4.3 kcal/mol lower. Moreover, the intermolecular mechanism has been ruled out by the crossover experiment (Fig. 5b ). Finally, Int V undergoes thermal conrotatory 4π-electrocyclization to give the product cis- thiirane II . Fig. 6: DFT calculation of the reaction mechanism via a thiocarbonyl ylide. Gibbs free energy profile at the M06-2X/6-311 + G(d,p)/PCM(DMF) level of theory. Full size image In summary, a generally applicable, highly stereoselective synthesis of cis -thiiranes has been realized under mild reaction conditions utilizing Lawesson’s reagent as a convenient sulfur source. 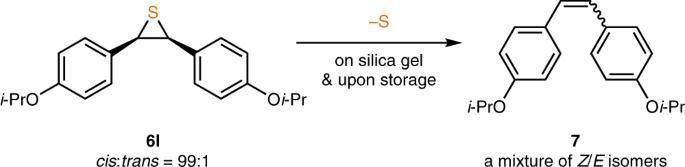Fig. 4: Instability of electron-rich thiirane. Non-stereospecific, spontaneous desulfurization ofp-alkoxy-cis-thiirane. 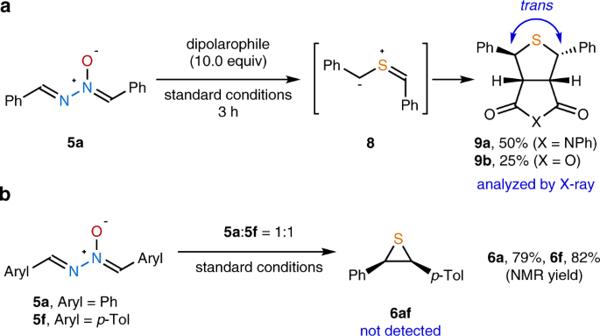Fig. 5: Mechanistic experiments. aTrapping thetrans-thiocarbonyl ylide intermediate with dipolarophiles.bCrossover experiment with two different aldazineN-oxides. 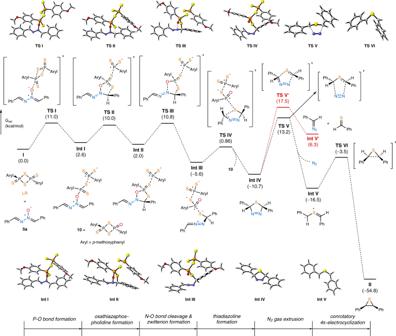Fig. 6: DFT calculation of the reaction mechanism via a thiocarbonyl ylide. Gibbs free energy profile at the M06-2X/6-311 + G(d,p)/PCM(DMF) level of theory. The newly developed method provides access to a wide variety of cis -1,2-diarylthiiranes from E , E -aldazine N- oxides in high yields with almost exclusive diastereoselectivity. Mechanistic experiments, as well as DFT calculation, suggest a reaction mechanism composed of stereospecific transformations involving 4π-electrocyclization of a trans -thiocarbonyl ylide as the origin of the exquisite diastereocontrol. Through this research, the useful sulfur congener of oxirane becomes available in a stereodefined form. Further expansion of this unique reactivity is currently investigated in our laboratories. A representative procedure for LR-mediated synthesis of cis -thiiranes from aldazine N -oxides To a mixture of benzaldazine N -oxide ( 5a , 224 mg, 1.00 mmol) in DMF (5.0 mL) was added LR (404 mg, 1.00 mmol) as a solution in DMPU (5.0 mL) at –50 °C dropwise under Ar. The change in internal temperature should not exceed 1 °C when the LR solution was added. After 4 h, the reaction mixture was transferred to a 100 mL separatory funnel and diluted with CH 2 Cl 2 (4 mL). The mixture was washed with water (50 mL × 3) and brine (50 mL). The combined aqueous layers were extracted with CH 2 Cl 2 (3 mL × 6). The combined organic layers were dried over anhydrous MgSO 4 (2 g), filtered through a glass frit, and concentrated in vacuo. The residue was purified immediately by flash column chromatography (SiO 2 , ø = 3.5 cm, l = 5.0 cm, hexanes, R f = 0.20, KMnO 4 ) to give cis -2,3-diphenylthiirane ( 6a , 165 mg, 78%, cis : trans = 99:1) as white solid. Data for 6a : 1 H NMR (400 MHz, CDCl 3 ): δ 7.14–7.10 (m, 10H), 4.38 (s, 2H); 13 C NMR (100 MHz, CDCl 3 ): δ 135.2, 129.5, 127.8, 127.3, 44.2; HRMS (ESI): [M–H] – calcd for C 14 H 11 S: 211.0587; found: 211.0586.